Global kinomic and phospho-proteomic analyses of the human malaria parasitePlasmodium falciparum The role of protein phosphorylation in the life cycle of malaria parasites is slowly emerging. Here we combine global phospho-proteomic analysis with kinome-wide reverse genetics to assess the importance of protein phosphorylation in Plasmodium falciparum asexual proliferation. We identify 1177 phosphorylation sites on 650 parasite proteins that are involved in a wide range of general cellular activities such as DNA synthesis, transcription and metabolism as well as key parasite processes such as invasion and cyto-adherence. Several parasite protein kinases are themselves phosphorylated on putative regulatory residues, including tyrosines in the activation loop of PfGSK3 and PfCLK3; we show that phosphorylation of PfCLK3 Y526 is essential for full kinase activity. A kinome-wide reverse genetics strategy identified 36 parasite kinases as likely essential for erythrocytic schizogony. These studies not only reveal processes that are regulated by protein phosphorylation, but also define potential anti-malarial drug targets within the parasite kinome. Malaria still kills over 1 million people a year and is a source of morbidity that represents a serious barrier to the social and economic progress of many second and third world countries [1] . Surprisingly, despite the fact that protein phosphorylation is a universal regulatory mechanism demonstrated as a druggable target in many human diseases, the potential of targeting the largely divergent protein kinases and phospho-signalling cascades of malaria parasites has been unexploited [2] , [3] . One of the factors contributing to this neglect is the serious paucity of information regarding the role played by phosphorylation in the biology of the most virulent human malaria parasite, Plasmodium falciparum . Two independent genomic analyses identified 86 (ref. 4 ) or 99 (ref. 5 ) genes encoding putative protein kinases in P. falciparum representing 1.1–1.6% of the coding genes, of which 65 are clearly related to the eukaryotic protein kinase (ePK) family. Many of the 65 P. falciparum ePKs can be assigned to the familiar AGC, CMGC, CK1, CaMK and tyrosine-kinase like groups observed in the human kinome [6] . In this respect the malarial and human kinomes are similar in that they are large and diverse gene families, which, certainly in the case of the human kinome, underlies multiple modes of regulation and diverse cellular substrates. Despite this overall similarity, however, sequence homology between malarial and mammalian protein kinases is limited in many instances, and as a consequence many Plasmodium protein kinases have no orthologues in the human host. These include the calcium-dependent kinases (CDPKs) that closely resemble plant kinases where the kinase domain is fused to a calmodulin-like domain [7] , and the FIKKs, which comprises the largest kinase family in P. falciparum with 21 members, and is restricted to Apicomplexan parasites [4] , [8] . Furthermore, there are some notably absent protein kinase classes in P. falciparum . In particular, there seems to be no members of the tyrosine kinase group, and no clearly recognizable MAPKK homologue, a family of the STE group. The significant phylogenetic diversity between the human and malarial kinomes could possibly provide the basis for selective targeting of the malarial kinome [2] . Although this is an attractive notion, there is very little information regarding the role of protein phosphorylation in Plasmodium biology, and hence predicting the potential efficacy and cellular effects of drugs targeting malarial kinases and phosphorylation pathways is difficult. It is in this light that we have combined kinome-wide gene knockout and reverse genetics approaches together with global phospho-proteomics to probe the importance of protein phosphorylation in the asexual intra-erythrocytic stages of P. falciparum . Our study shows that ∼ half of the 65 ePKs that make up the P. falciparum kinome are likely to be essential for the maintenance of parasite viability. This surprising lack of redundancy points not only to the pivotal role of a number of individual protein kinases but also to a potentially abundant source of anti-malarial protein kinase targets. That these protein kinases regulate a diverse range of biological activities is evident by the nature of the phospho-proteome, which we show here includes proteins involved in many key processes such as invasion into red blood cells, metabolism, transcription and DNA replication. The complexity of protein phosphorylation in malaria parasites was further underlined by our observation that despite the absence of a classical tyrosine kinase family in P. falciparum , tyrosine phosphorylation does indeed occur in the parasite. This is exemplified by the protein kinase PfCLK3 (PF11_0156), which is phosphorylated on tyrosine within the activation loop in a manner consistent with this kinase being a member of the dual-specificity tyrosine phosphorylated-regulated kinase (DYRK) family. Kinome-wide reverse genetics in P. falciparum To identify protein kinases that are essential for asexual proliferation, and hence represent potential targets for curative intervention, we attempted to inactivate each of the entire complement of 65 ePK genes that constitute the P. falciparum kinome [4] (this study does not include FIKKs, a novel divergent, Apicomplexa-specific kinase-like family we identified in our initial kinome analysis). This was achieved following a homologous recombination, single crossover gene disruption strategy ( Supplementary Figs S1-S3 ). Integration of the KO vectors into the genome of transfected parasites (clone 3D7) was monitored by PCR and/or Southern blot analysis ( Supplementary Fig. S4 ). 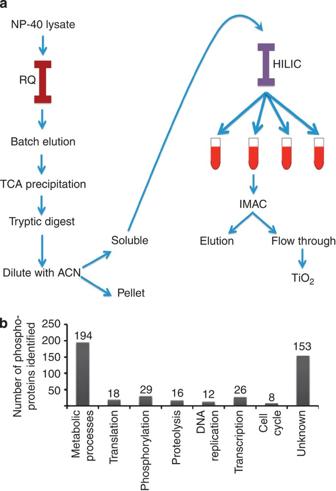Figure 1: Global phospho-proteomic analysis of the schizont stage ofP. falciparum. (a) Schematic illustration of the protocol of tryptic phospho-peptide preparation and enrichment from a 1% NP-40 lysate of the schizont stage (36–40 h) ofP. falciparum. This protocol was conducted on six biological replicates to generate the list of phosphorylation sites summarized in this figure and detailed in theSupplementary Data 1and2. (ACN; acetonitrile, IMAC; immobilised metal affinity chromatography, TiO2; titanium dioxide). (b) Histogram representing fractional distribution of functionally different groups of parasite phospho-proteins. Uniprot accessions of the identifiedPlasmodium falciparumphospho-proteins were imported into Blast2GO and Blast searching was carried out against the NCBI non-redundant protein database. Gene Ontology mapping and further annotation were performed using default Blast2GO parameters. Integration of the KO vector was not observed after a prolonged (at least 90 days) culture for 27 ePK genes, indicating that the enzymes encoded by these genes likely have crucial roles in parasite asexual proliferation ( Table 1 ). For the majority (22) of these 27 loci, we separately transfected 3D7 parasites with tagging vectors designed to place a C-terminal tag (haemagglutinin, Myc or green fluorescent protein) in-frame with the ePK coding sequence ( Supplementary Fig. S1 ). In all cases except PfPK6 (PF13_0206) and PfCLK3 (PF11_0156), targeting of the locus with the epitope tag was successful ( Table 1 , Supplementary Fig. S1 ; Supplementary Table S1 ); the lack of success in tagging PfPK6 and PfCLK3 may reflect a deleterious effect of the tag on enzyme function. For 3 of the 27 genes that could not be disrupted by the KO vector alone (PfCK2 (PF11_0096), PfPK9 (PF13_0085) and Pfmap-2 (PF11_0147)), we were able to achieve gene disruption if the function was complemented through co-transfection of the ePK of interest under the control of the P. falciparum Hsp86 promoter ( Table 1 , Supplementary Fig. S2 ). This complementation approach can now be applied for detailed functional investigations of these enzymes, for example, by examining the effect of specific mutations in the complementing gene, notably gatekeeper residue mutations that confer hypersensitivity to bulky inhibitors (see below). Table 1 PKs considered as likely essential for the erythrocyte asexual cycle. Full size table Taken together, the tagging and complementation approaches strongly suggest that for 22 ePKs the absence of integration of the KO vector is not caused by locus refractoriness to recombination but rather is likely due to the fact that these ePKs have a crucial role in the erythrocytic asexual cycle, the process that is responsible for malaria pathogenesis. Among these 22 ePKs are 8 enzymes that we previously reported as playing a crucial role in asexual proliferation: Pfmap-2 (PF11_0147) [9] , Pfnek-1 (PFL1370w) [10] , PfCK2 (PF11_0096) [11] , PfTKL3 (PF13_0258) [12] , Pfcrk-3 (PFD0740w) [13] , PfCLK1 (PF14_0431) [14] , PfCLK2 (PF14_0408) [14] and PfARK1 (PF13_0258) [15] . Others have provided reverse genetics evidence for essentiality of three additional ePKs, PfCDPK1 (PFB0815w) [16] , PfPKG (PF14_0346) [17] and PfPCDPK5 (PF13_0211) [18] . Hence, the present study brings to 25 the number of ePKs that are highly likely to have a crucial role in the erythrocytic asexual cycle of P. falciparum (highlighted in bold in Table 1 ). In contrast, we detected integration of the KO vector into the gene loci of 32 ePKs. In six cases (indicated by flanking asterisks in Table 1 ), the signals were very weak even after prolonged culture; we propose that the weak PCR signal diagnostic for integration of the KO vector indicates that integration occurs transiently during schizogony but that parasites with a disrupted locus do not persist. We consider these genes are likely to be essential; genotyping of cloned populations will be required to validate this interpretation for this subset of ePK genes. In the case of one of these kinases, the cyclic AMP (cAMP)-dependent kinase PfPKA, an essential role is further supported by the observation that transgenic parasites expressing mutant cAMP-dependent phosphorylation sites in the apical membrane antigen 1 protein are significantly impaired in the invasion process [19] . 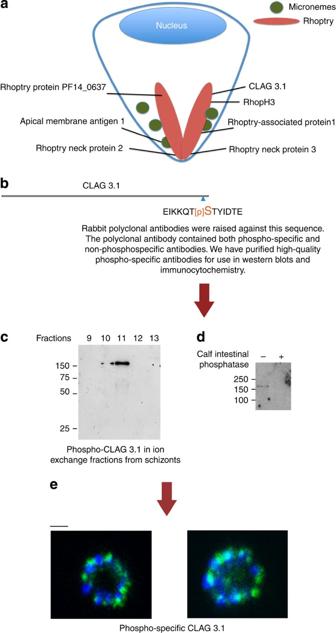Figure 2: Phosphorylation status of microneme and rhoptry proteins. (a) Schematic summary of the rhoptry and microneme phospho-proteins. (b) Illustration of the sequence to which phospho-specific CLAG 3.1 antibodies were raised. (c) Lysates from schizont stage-infected RBCs were fractionated on an RQ ion exchange column. A sample from each fraction was resolved by SDS-polyacrylamide gel electrophoresis and the gel probed with anti-phospho CLAG 3.1 antibody. Shown are the results from fractions 9 to 13 from the RQ column elution. (d) To determine if the antibody recognized the phosphorylated form of CLAG 3.1, fraction 11 from the RQ column was treated with calf intestinal phosphatase to remove all phosphorylation. Control samples were not treated with phosphatase. The fraction was then probed with the anti-phospho CLAG 3.1 antibody. (e) The anti-phospho-CLAG 3.1 antibody was used to determine the localization of phospho-CLAG 3.1 by immunocytochemistry of paraformaldehyde-fixed schizont stage parasites. Shown are two examples of schizont (segmenter) parasites stained with the phospho-CLAG 3.1 antibody. The samples were also stained with 4,6-diamidino-2-phenylindole (blue) to label the nuclei. The scale bar indicates 2 μM. The experiments shown are representative of at least three independent experiments. For 25 ePKs genes, a strong signal was obtained for integration of the KO vector in transfected populations, suggesting that the products of these genes are not essential for completion of the asexual intra-erythrocytic cycle, or that other protein kinases can compensate for the inactivated gene ( Table 2 ). This was firmly established for 12 of these, for which parasite clones with a disrupted locus were obtained by limited dilution. In addition, PfCDPK4 (PF07_0072) was previously identified by Kato et al . [16] as being dispensable for asexual growth. Table 2 PKs considered as likely dispensable for the erythrocyte asexual cycle. Full size table In summary, our initial assessment of essential function indicates that of the 65 ePks in the P. falciparum kinome, 36 ePKs are likely to have a crucial role in the P. falciparum erythrocytic asexual cycle ( Table 1 ). In contrast, 12 are definitely dispensable, as evidenced by viable parasite clones in which the relevant genes are inactivated (indicated in bold in Table 2 ) and a further 14 are likely dispensable (indicated by flanking asterisks in Table 2 ). Global phospho-proteome of P. falciparum In order to provide a comprehensive picture of the malarial phospho-proteome we undertook a mass spectrometry-based global phospho-proteomic study of the late schizont stage of P. falciparum . Following lysis of purified schizonts in 1% NP-40 the entire infected red blood cell extract was processed as summarized in Figure 1a . This process identified 676 phosphoproteins, of which 26 were human proteins and 650 were from the parasite ( Supplementary Data 1 and 2 ). In total we identified 1223 individual phosphorylation sites, the vast majority of which (1177) occurred on proteins encoded by the parasite ( Fig. 1b ). Supplementary Data 1 and 2 provide a full list of human and parasite phospho-proteins and phospho-sites, respectively. The phospho-peptides presented in these spread sheets have been observed in at least two of the six biological replicates analysed and were derived from a total data set of 3289 unique phospho-peptides which were filtered using stringent criteria that included computational analysis and manual inspection of each MS/MS spectrum (see Supplementary Methods ). A SCAFFOLD file containing all the MS/MS data from this study can be downloaded as described in the methods section. Figure 1: Global phospho-proteomic analysis of the schizont stage of P. falciparum . ( a ) Schematic illustration of the protocol of tryptic phospho-peptide preparation and enrichment from a 1% NP-40 lysate of the schizont stage (36–40 h) of P. falciparum . This protocol was conducted on six biological replicates to generate the list of phosphorylation sites summarized in this figure and detailed in the Supplementary Data 1 and 2 . (ACN; acetonitrile, IMAC; immobilised metal affinity chromatography, TiO2; titanium dioxide). ( b ) Histogram representing fractional distribution of functionally different groups of parasite phospho-proteins. Uniprot accessions of the identified Plasmodium falciparum phospho-proteins were imported into Blast2GO and Blast searching was carried out against the NCBI non-redundant protein database. Gene Ontology mapping and further annotation were performed using default Blast2GO parameters. Full size image In addition to the identification of phospho-proteins involved in general cellular activities such as metabolism, DNA replication and gene transcription ( Fig. 1b ), many of the phospho-proteins were associated with parasite-specific processes such as cyto-adhesion (for example, knob-associated histidine-rich protein (PFB0100c)), a process that is central to malaria pathogenesis ( Supplementary Data 2 ). Parasite invasion into red blood cells is a complex process involving merozoite binding, reorientation, shedding of merozoite coat proteins and invasion per se [20] . We show here that proteins involved in this process are phosphorylated including the microneme protein apical membrane antigen 1 (PF11_0344) ( Fig. 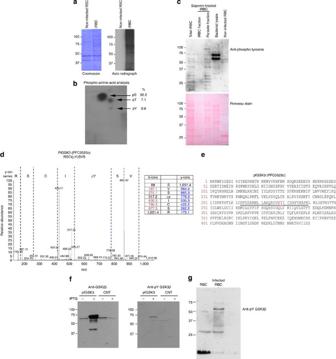Figure 3: Determination of tyrosine phosphorylation inP. falciparumincluding tyrosine phosphorylation of PfGSK3. (a) 106Human RBCs or the same number for infected schizont stage RBCs were labelled with [32P]-orthophosphate. The cells were then lysed in 1%NP-40 lysis buffer and the sample was resolved by SDS-polyacrylamide gel electrophoresis (PAGE). Before an autoradiograph was obtained (right panel) the gel was stained with coomassie blue (left panel). (b) The lysate from metabolically labelled schizont stage parasites was also processed for analysis of the phospho-amino acids. Shown is an autoradiograph from such an experiment where the positions of phosphorylated amino-acid standards are indicated. The spots corresponding to each of the standards were scrapped and the radioactive content determined by liquid scintillation counting. The relative amounts of radioactivity associated with each phospho-amino acid were then calculated. Shown is a representative result from three independent experiments. (c) Schizont stage-infected RBCs were either lysed in 1% NP-40 to give total iRBC sample or fractionated into a RBC fraction (iRBC fraction) or parasite fraction following saponin lysis. Controls were bacterial lysates and non-infected RBC lysates. The samples (20 μg) were resolved by SDS-PAGE and the gels probed in a western blot using an anti-phospho tyrosine antibody. To determine the loading of proteins, gels were stained with Ponceau stain. (d) An example of a typical LC-MS/MS trace identifying phosphorylation at Y229within the activation loop of PfGSK3. (e) Sequence of PfGSK3 showing the activation loop (underlined) and the position of phospho-Y229highlighted in red. (f) Bacteria transformed with an expression plasmid containing either PfGSK3 or as a control PfCK2α (CNT) were either induced or non-induced with IPTG. These bacteria were lysed and the extract (20 μg) was used in western blots probed with antibodies against the human GSK3α/β (left panel) or an antibody against human tyrosine-phosphorylated GSK3α/β-pY279/216(right panel). (g) Confirmation of the phosphorylation of PfGSK3 at Y229in a western blot using a commercial antibody against the tyrosine phosphorylation site on human GSK3α/β-pY279/216. Lysates (20 μg) were obtained from 106infected RBCs or the same number of non-infected RBCs (as a control). The experiments shown are representative of at least three independent experiments. 2a , Table 3 ), a protein whose phosphorylation was previously shown to be important for invasion [19] , and the merozoite cell surface proteins MSP1 and MSP7 ( Supplementary Data 2 ), together with proteins associated with the rhoptries, specialized organelles at the apical pole of merozoites that release proteins during the invasion process [21] ( Fig. 2a , Table 3 ). The phosphorylation status of one of these rhoptry proteins, CLAG 3.1, that forms part of the RhopH complex proposed to have a role in erythrocyte binding [21] , formation/function of the parasitophorous vacuole [21] , [22] , cyto-adherence [23] and invasion [21] , was confirmed using an anti-phospho antibody raised against pS 1382 ( Fig. 2b–d ). This antibody identified a punctuate localization of phospho-CLAG 3.1 consistent with rhoptry localization within merozoites of a mature schizont ( Fig. 2e ). A recent report implicating CLAG3.1 in the machinery that imports nutrient in the infected red blood cell [24] suggests that phosphorylation may also regulate this process, which is fundamental in parasite survival. Figure 2: Phosphorylation status of microneme and rhoptry proteins. ( a ) Schematic summary of the rhoptry and microneme phospho-proteins. ( b ) Illustration of the sequence to which phospho-specific CLAG 3.1 antibodies were raised. ( c ) Lysates from schizont stage-infected RBCs were fractionated on an RQ ion exchange column. A sample from each fraction was resolved by SDS-polyacrylamide gel electrophoresis and the gel probed with anti-phospho CLAG 3.1 antibody. Shown are the results from fractions 9 to 13 from the RQ column elution. ( d ) To determine if the antibody recognized the phosphorylated form of CLAG 3.1, fraction 11 from the RQ column was treated with calf intestinal phosphatase to remove all phosphorylation. Control samples were not treated with phosphatase. The fraction was then probed with the anti-phospho CLAG 3.1 antibody. ( e ) The anti-phospho-CLAG 3.1 antibody was used to determine the localization of phospho-CLAG 3.1 by immunocytochemistry of paraformaldehyde-fixed schizont stage parasites. Shown are two examples of schizont (segmenter) parasites stained with the phospho-CLAG 3.1 antibody. The samples were also stained with 4,6-diamidino-2-phenylindole (blue) to label the nuclei. The scale bar indicates 2 μM. The experiments shown are representative of at least three independent experiments. Full size image Table 3 Summary of rhoptry and microneme phospho-peptides and phospho-proteins observed in the schizont stage of P. falciparum -infected red blood cells. 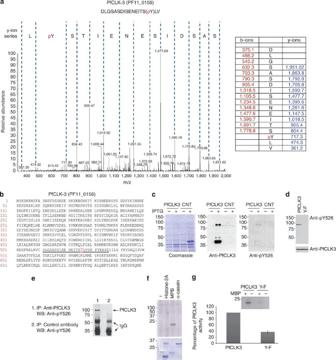Figure 4: Tyrosine phosphorylation of PfCLK3. (a) An example of a typical LC-MS/MS trace identifying phosphorylation at Y526within the activation loop of PfCLK3. (b) Sequence of PfCLK3 showing the activation loop (underlined) and the position of phospho-Y526highlighted in red. (c) Bacteria transformed with an expression plasmid containing either PfCLK3 or as a control PfPKA (CNT) were either induced or non-induced with IPTG. These bacteria were lysed and the extract (20 μg) was used in western blots probed with structural antibodies against the PfCLK3 (middle panel) or antibodies against tyrosine 526 on PfCLK3 (right hand panel). The coomassie stain of the samples is shown as a loading control on the left. (d) Bacterially expressed PfCLK3 or a mutant of PfCLK3 where Y526was mutated to a phenylalanine (Y-F) was purified and resolved by SDS-polyacrylamide gel electrophoresis. The gel was probed in a western blot with antibodies against tyrosine 526 on PfCLK3 (anti-pY526) or as a loading control structural antibodies against the PfCLK3 (anti-PfCLK3). (e) Saponin-treated schizont parasite extract was immunoprecipitated with structural antibodies against the PfCLK3 (Anti-PfCLK3) or control immunoglobulin G (antibodies to an unrelated protein the M1-muscarinic receptor). The immunoprecipitate was then probed in a western blot with antibodies against tyrosine 526 on PfCLK3 (anti-pY526). (f) The activity of purified bacterially expressed PfCLK3 was determined inin vitrokinase assays containing either no substrates or Histone 2A, myelin basic protein (MBP) or α-casein. Shown is a representative autoradiograph of the phosphorylated substrates with a coomassie stain of the same gel as a loading control. (g) Purified bacterially expressed PfCLK3 or a mutant of PfCLK3 where Y526was mutated to a phenylalanine (Y-F) (0.5 μg) was used in anin vitrokinase assays with myelin basic protein (MBP) as a substrate. Shown is a representative autoradiograph and below the cumulative mean data of three independent experiments±s.d. (n=3). Full size table Activation loop threonine phosphorylation of parasite protein kinases The global phospho-proteomic study revealed that at least 23 protein kinases are phospho-proteins ( Table 4 ) and that a number of these phosphorylation events occurred within the activation loop, a process that is often necessary for the full activation of protein kinases [25] . These included activation loop phosphorylation of T 189 on PfPKA (PFI1685w) and T 695 on PfPKG (PF14_0346) in a manner that resembles activation loop phosphorylation in the mammalian orthologues, which is necessary for full kinase activity. These phosphorylation sites were confirmed in a phospho-proteomic study conducted by Drs Edwin Lasonder and Pietro Alano (personal communication), and by western blot experiments using anti-phospho T 189 antibodies to PfPKA and anti-phospho T 695 antibodies to PfPKG ( Supplementary Fig. S5 ). Table 4 Summary of parasite protein kinases and kinase regulatory proteins that were observed as phospho-proteins in the schizont stage of P. falciparum -infected red blood cells. Full size table The essential P. falciparum cyclin-dependent protein kinases Pfcrk-1 (PFD0865c) and Pfcrk-3 (PFD0740w) ( Table 1 ) are also phosphorylated on threonine residues within the activation loop. This may well represent dynamic/regulatory phosphorylation analogous to that observed for the mammalian and fungal cyclin-dependent kinases (CDKs) that require both cyclin binding and the activation loop threonine phosphorylation for full activity [26] . In the case of the mammalian CDKs, this phosphorylation is mediated through a CDK-activating kinase. A good candidate for such a kinase acting upstream of Pfcrk-1 and Pfcrk-3 in P. falciparum would be Pfmrk (PF10_0141), a CDK that displays closest homology to CDK-7, the CDK-activating kinase mammalian homologue. Activation loop tyrosine phosphorylation of parasite protein kinases Despite the lack of a recognized tyrosine kinase family [27] in the P. falciparum kinome, phospho-amino acid analysis of metabolically labelled schizonts revealed trace amounts of phospho-tyrosine (<1% of total protein phosphorylation) ( Fig. 3a,b ). Furthermore, using anti-phosphotyrosine antibodies we demonstrated that infected red blood cells (RBCs) undergo a substantial increase in tyrosine phosphorylation over non-infected controls, and that the majority of this tyrosine phosphorylation was detectable within the parasite fraction ( Fig. 3c ). It seems therefore that tyrosine phosphorylation may occur within the parasitophorous vacuole (including within the parasite itself) rather than exclusively in the host erythrocyte. Figure 3: Determination of tyrosine phosphorylation in P. falciparum including tyrosine phosphorylation of PfGSK3. ( a ) 10 6 Human RBCs or the same number for infected schizont stage RBCs were labelled with [ 32 P]-orthophosphate. The cells were then lysed in 1%NP-40 lysis buffer and the sample was resolved by SDS-polyacrylamide gel electrophoresis (PAGE). Before an autoradiograph was obtained (right panel) the gel was stained with coomassie blue (left panel). ( b ) The lysate from metabolically labelled schizont stage parasites was also processed for analysis of the phospho-amino acids. Shown is an autoradiograph from such an experiment where the positions of phosphorylated amino-acid standards are indicated. The spots corresponding to each of the standards were scrapped and the radioactive content determined by liquid scintillation counting. The relative amounts of radioactivity associated with each phospho-amino acid were then calculated. Shown is a representative result from three independent experiments. ( c ) Schizont stage-infected RBCs were either lysed in 1% NP-40 to give total iRBC sample or fractionated into a RBC fraction (iRBC fraction) or parasite fraction following saponin lysis. Controls were bacterial lysates and non-infected RBC lysates. The samples (20 μg) were resolved by SDS-PAGE and the gels probed in a western blot using an anti-phospho tyrosine antibody. To determine the loading of proteins, gels were stained with Ponceau stain. ( d ) An example of a typical LC-MS/MS trace identifying phosphorylation at Y 229 within the activation loop of PfGSK3. ( e ) Sequence of PfGSK3 showing the activation loop (underlined) and the position of phospho-Y 229 highlighted in red. ( f ) Bacteria transformed with an expression plasmid containing either PfGSK3 or as a control PfCK2α (CNT) were either induced or non-induced with IPTG. These bacteria were lysed and the extract (20 μg) was used in western blots probed with antibodies against the human GSK3α/β (left panel) or an antibody against human tyrosine-phosphorylated GSK3α/β-pY 279/216 (right panel). ( g ) Confirmation of the phosphorylation of PfGSK3 at Y 229 in a western blot using a commercial antibody against the tyrosine phosphorylation site on human GSK3α/β-pY 279/216 . Lysates (20 μg) were obtained from 10 6 infected RBCs or the same number of non-infected RBCs (as a control). The experiments shown are representative of at least three independent experiments. Full size image The clearest example of tyrosine-phosphorylated parasite proteins emerging from the global phosphorylation analysis was tyrosine phosphorylation of parasite protein kinases within the activation loop. Tyrosine 229 within the activation loop of P. falciparum glycogen synthase kinase 3 (PfGSK3) (PFC0525c), an enzyme that is likely essential for asexual proliferation ( Table 1 ), was observed to be phosphorylated ( Fig. 3d–g ). This site is analogous to Y 279 and Y 216 on mammalian GSK3α/β, the activation loop auto-phosphorylation sites necessary for enzymatic activity [28] . We exploited the fact that antibodies to human GSK3α/β (pY 276/216 ) cross-react with PfGSK3 ( Fig. 3f ) to confirm that PfGSK3 was indeed phosphorylated on Y 229 at the schizont stage ( Fig. 3g ). Furthermore, we showed that PfGSK3 expressed as a recombinant protein in bacteria was also phosphorylated on Y 229 ( Fig. 3f ), suggesting that this phosphorylation event arises by auto-phosphorylation, as observed for mammalian GSK3α/β [28] . Further tyrosine phosphorylation was detected within the activation loop of the P. falciparum protein kinase PfCLK3 (PF11_0156) ( Fig. 4a,b ), which is also likely to be an essential kinase ( Table 1 ) and is related to the pre-mRNA processing kinase hPRP4 found in higher eukaryotes [4] . Phylogenetic analysis shows that these two kinases belong to a cluster that also includes the DYRKs sub-family [4] , [29] . The DYRKs are serine/threonine kinases of the CMGC kinase family that are characterized by the formation of an active transient intermediate during translation that is able to catalyse cis-auto-phosphorylate on tyrosine [29] , [30] . This process is proposed to be essential for full catalytic activity of the mature form of the enzyme, which then shows only serine/threonine kinase activity. Unlike most DYRKs that have a YXY motif in the activation loop where the second Y is the site of auto-phosphorylation [29] , PfCLK3 contains an TSY motif in the same position. The global phosphorylation study determined that tyrosine 526 within this motif in PfCLK3 was phosphorylated in vivo ( Fig. 4a,b ), an observation confirmed by using an anti-phosphopeptide antibody against pY 526 ( Fig. 4c,d ) that was able to identify pY 526 on PfCLK3 immunoprecipitated from schizont stage-infected red blood cells ( Fig. 4e ). Figure 4: Tyrosine phosphorylation of PfCLK3. ( a ) An example of a typical LC-MS/MS trace identifying phosphorylation at Y 526 within the activation loop of PfCLK3. ( b ) Sequence of PfCLK3 showing the activation loop (underlined) and the position of phospho-Y 526 highlighted in red. ( c ) Bacteria transformed with an expression plasmid containing either PfCLK3 or as a control PfPKA (CNT) were either induced or non-induced with IPTG. These bacteria were lysed and the extract (20 μg) was used in western blots probed with structural antibodies against the PfCLK3 (middle panel) or antibodies against tyrosine 526 on PfCLK3 (right hand panel). The coomassie stain of the samples is shown as a loading control on the left. ( d ) Bacterially expressed PfCLK3 or a mutant of PfCLK3 where Y 526 was mutated to a phenylalanine (Y-F) was purified and resolved by SDS-polyacrylamide gel electrophoresis. The gel was probed in a western blot with antibodies against tyrosine 526 on PfCLK3 (anti-pY526) or as a loading control structural antibodies against the PfCLK3 (anti-PfCLK3). ( e ) Saponin-treated schizont parasite extract was immunoprecipitated with structural antibodies against the PfCLK3 (Anti-PfCLK3) or control immunoglobulin G (antibodies to an unrelated protein the M1-muscarinic receptor). The immunoprecipitate was then probed in a western blot with antibodies against tyrosine 526 on PfCLK3 (anti-pY526). ( f ) The activity of purified bacterially expressed PfCLK3 was determined in in vitro kinase assays containing either no substrates or Histone 2A, myelin basic protein (MBP) or α-casein. Shown is a representative autoradiograph of the phosphorylated substrates with a coomassie stain of the same gel as a loading control. ( g ) Purified bacterially expressed PfCLK3 or a mutant of PfCLK3 where Y 526 was mutated to a phenylalanine (Y-F) (0.5 μg) was used in an in vitro kinase assays with myelin basic protein (MBP) as a substrate. Shown is a representative autoradiograph and below the cumulative mean data of three independent experiments±s.d. ( n =3). Full size image That this phosphorylation on PfCLK3 was likely to be due to auto-phosphorylation was evidenced by the fact that bacterially expressed PfCLK3 was phosphorylated on tyrosine 526 ( Fig. 4c ). Furthermore, we determined that bacterially expressed PfCLK3 was able to phosphorylate myelin basic protein in vitro ( Fig. 4f ). Using this assay we probed the importance of pY 526 phosphorylation and determined that PfCLK3 activity was reduced by ∼ 60% following mutation of the Y 526 -F ( Fig. 4g ). These findings are consistent with the notion that this protein kinase is a DYRK. Hence, our data point to constitutive auto-phosphorylation of PfCLK3 at tyrosine 526 being important for enzymatic activity but that further regulation by either controlling expression levels, subcellular localization or via additional phosphorylation outside the activation loop may also be in operation to fine tune PfCLK3 kinase activity. In addition to ePK activation loops, our phosphoproteome also detected tyrosine phosphorylation on a small number of non-kinase proteins that are located within the parasite, such as the DNA-replicating factor PfMCM2 (PF14_0177). These tyrosine-phosphorylated proteins were, however, only observed in one biological replicate and as such are not included in Supplementary Data 2 (although they are present in the SCAFFOLD file). The fact that we only saw these tyrosine phospho-peptides once might be due to the extremely low abundance of tyrosine-phosphorylated proteins as indicated from the phospho-amino acid analysis ( Fig. 3b ). The presence of these rare peptides does, however, suggest that some of the parasite's serine/threonine protein kinase/s possess dual specificity and are able to also phosphorylate tyrosine residues, as has been established in other ePKs, for example protein kinase CK2 [31] . We are currently investigating this possibility. The reverse genetics study we present here attempts to determine which of the parasite ePKs are required for completion of the asexual cycle in erythrocytes. Interestingly, comparing Tables 1 and 2 indicates that the various ePK groups and families are not distributed evenly between the essential and non-essential kinases. For example, almost all the CMGC group kinases and all aurora-related kinases seem to be essential for the asexual cycle, whereas 3 out of 4 NimA-related kinases are dispensable, illustrating the different requirements for specific functions at distinct stages of the life cycle. Formal demonstration of non-essentiality requires genotyping of clonal lines, which at present has been achieved for 12 of the 26 ePKs genes in Table 2 ( Supplementary Table S1 and Supplementary Fig. S3 for a specific example). Although it is highly likely that the remaining 14 kinases (those highlighted with asterisks in Table 2 ) are dispensable for asexual growth, definitive demonstration of this awaits the generation and genotyping of cloned populations. Although most parasites with an inactivated ePK gene did not show any obvious growth defects, we observed two instances (PfPK7 (PFB0605w) [32] and Pfcrk-5 (PFF0750w)) where the ePK disruptants showed a slow parasitemia growth curve (typical growth curves are displayed in Supplementary Figs S6 and S7 ) in addition to genotyping data for these two genes); a detailed study of the PfPK7 KO phenotype has been published [32] . There may be additional kinases whose deletion causes a growth phenotype; comprehensive evaluation in this respect has to await availability of clones for all instances where gene disruption has been achieved. Two of the dispensable ePKs, PfeIK1 and PfeIK2, are from the 'eukaryotic initiation factor 2α kinase' family. PfeIK1 is expressed in asexual parasites, and was shown to be required for starvation-dependent phosphorylation of PfeIF2α during the erythrocytic cycle [33] whereas PfeIK2 is expressed predominantly during sexual development and is required to prevent premature translation of liver stage-specific genes in salivary gland sporozoites [34] . Interestingly, the third eIF2α kinase in the P. falciparum kinome, PfPK4, seems to be essential for asexual growth. If its function is indeed to prevent general translation through phosphorylation of PfeIF2α (as suggested by its ability to phosphorylate an eIF2α peptide in vitro [35] ), it follows that translation inhibition through phosphorylation of the translation factor is an essential feature at some stage of the erythrocytic asexual cycle. A testable hypothesis is that this happens at late stages of merozoite ontogeny and in mature merozoites, the only stages of the cycle where translation is essentially inactive. Noteworthy is the fact that none of the available parasite clones with a disrupted kinase gene that have been examined thus far display an obvious phenotype in the rate of gametocytogenesis; until we have cloned and phenotyped all populations with a disrupted gene, we cannot of course exclude the possibility that one of these enzymes is required for gametocytogenesis. If a specific kinase regulates commitment to gametocytogenesis but is also required for (an)other function(s) essential for asexual growth, uncovering the former will require conditional expression or activity of the 36 kinases that are classed in this study as 'likely essential'. Some of the ePKs that are not essential for asexual growth have already been demonstrated to be required for successful infection of the mosquito vector [32] , [36] ; in light of this we are currently aiming to phenotype KO clones of all non-essential ePKs in the mosquito. Our data indicate that a total of 36 ePKs ( Table 1 ) are likely to have an essential role in the P. falciparum erythrocytic asexual cycle and that 26 ePKs are likely to be dispensable ( Table 2 ). In comparison, a recent study of 66 ePKs of the rodent malaria parasite P. berghei identified 43 protein kinases that are refractory to deletion in the blood stage and 23 whose genes could be deleted [37] ( Supplementary Table S1 ). Although there is overall a good level of agreement between the ePKs identified as essential in the mouse parasite and those we identify here to be have a crucial role in P. falciparum ( Supplementary Table S1 ), there are nevertheless differences, which may underlie divergence between human and mouse malarial species resulting from a split estimated to have occurred 70 million years ago. We emphasise here that formal demonstration that a given ePK gene is not essential for asexual schizogony requires analysis of clones from the populations displaying evidence for gene disruption or deletion; this has been achieved for the entire P. berghei kinome [37] but thus far only partially in P. falciparum . Overall, the phospho-proteomic analysis reported here demonstrates that protein phosphorylation is widely employed in the regulation of cellular processes within the asexual blood stage of P. falciparum . This not only includes general house-keeping functions such as metabolism, DNA replication and transcription but also parasite-specific processes such as red blood cell invasion and cyto-adherence. Furthermore, the identification of tyrosine phosphorylation within the activation loop of essential protein kinases presents evidence for tyrosine phosphorylation being important in the viability of the blood stage parasite. The importance of protein phosphorylation in the viability of the human malaria parasite is further supported by the fact that ∼ half of the parasite ePKs are likely to be essential for the blood stage parasites. Thus, the extensive phospho-proteome together with the lack of redundancy among many of the ePKs supports the notion that targeting parasite protein phosphorylation at the blood stage may represent an effective strategy for the treatment of P. falciparum infection. One of the major drawbacks of targeting protein kinases in human disease is the fact that selective inhibitors are considered difficult to generate due to the fact that many inhibitors target the conserved ATP-binding site [38] . It is, however, possible to build selectivity into ATP-competitive inhibitors by extending the interaction of the inhibitor molecules to non-conserved allosteric sites located within a hydrophobic pocket adjacent to the ATP-binding site [38] , [39] . This strategy has been successfully employed for a number of protein kinase inhibitors designed to target human kinases in the treatment of cancer [40] including the clinically approved Bcr–Abl inhibitor Imatinib (Gleevec) [41] . That a similar approach to drug design may be effective in the search for molecules with selectivity against malaria is supported by the significant phylogenetic diversity between the human and plasmodial kinomes [4] . Such a strategy relies on the pharmacological compounds obtaining access to the allosteric sites. This is determined primarily by a gatekeeper residue situated on the β5 strand of region V, which is distal to the active site and adjacent to the hinge region. If the gatekeeper residue is bulky (for example, phenylalanine) then access to the allosteric sites are blocked, whereas a small (for example, threonine) or even a medium-sized (methionine) gatekeeper residue would allow access [38] . Importantly, of the 36 protein kinases determined likely to be essential for the blood stage 4 have a small gatekeeper residue (threonine) and 11 have a medium-sized gatekeeper (methionine). Exploiting the accessibility of the allosteric sites within these enzymes provides a strategy for the development of selective parasite protein kinase inhibitors with parasiticidal activity. It is possible that one source of these novel kinase inhibitors may be found within recent screening programmes that have identified thousands of chemical entities with anti-malarial activity, many of which have chemo-forms consistent with protein kinase inhibitors [42] . Mining the results of these screens to identify drug-like compounds that target essential parasite protein kinases and phosphorylation pathways might provide a potential route to the next generation of anti-malarials. Accessing the phospho-proteomic data All of the manually validated phospho-peptides observed in this study are listed in Supplementary Data 1 and 2 . In addition we have made available the SCAFFOLD file containing all the mass spectrometry data associated with this manuscript. This may be downloaded from https://proteomecommons.org , using the following Tranche hash: JtHgFyh9HqIYMNWlXk2BTxavNlZutqY1fwalNMWAxEu7GmsuVFw0xQzUAuGf/3ZKgnXmZb33 wtuawOhR33cSO0QY2TsAAAAAAAAEvA== To view the SCAFFOLD file it will be necessary to download the SCAFFOLD viewer, which is free from the following site http://www.proteomesoftware.com/ Construction of knockout plasmids For each ePK, a fragment from the open reading frame (typically ∼ 500 bp in length) was amplified by PCR and inserted between the BamHI and NotI sites of the pCAM-BSD plasmid [43] which contains the Aspergillus terrus blasticidine-S-deaminase gene, whose gene product confers resistance to the drug Blasticidin. Cloning primers are listed in Supplementary Data 3 . Construction of the complementation plasmids Plasmids for in vivo episomal expression of selected ePKs (see Table 1 ) were constructed as follows: the full-length coding sequence was first inserted between the BglII and NotI sites of the plasmid pHGB [44] and then transferred into the plasmid pCHD-1/2 by a Gateway LR clonase reaction according to the manufacturer's instructions (Invitrogen). The plasmid pCHD-1/2 includes a cassette-encoding hDHFR, conferring resistance to the antifolate drug WR99210. Parasites that were transfected with both a knockout plasmid and a complementation plasmid were cultured under double drug selection ( Supplementary Methods ). Phospho-amino acid analysis Magnetic cell sorting-purified iRBC ( ∼ 50 μl pellet volume) were resuspended in 500 μl Krebs buffer (phosphate free) and incubated with 20–25 μl fresh 32 P-orthophosphate for 30 min at 37 °C. Following incubation the pellet was washed twice with 1 ml PBS containing protease and phosphotase inhibitors (Roche) and lysed with lysis buffer: 50 mM Tris, 0.5 mM EDTA, 5% β-glycerophosphate, pH7.6, supplemented with protease/phosphatase inhibitors (Roche) and 1% NP-40. The lysate was prepared and purified by means of 2-D Clean-Up Kit (Amersham Biosciences) following the manufacturer's instructions. Final pellets were briefly air dried and resuspended in 20 μl 6 M HCl and immediately placed in preheated to 110 °C oven for hydrolysis. After 1 h hydrolysis samples were cooled down to room temperature, resuspended in 400 μl H 2 O and spun 5 min at 21,000 g . The supernatant fractions were dried at 30 °C on a speedvac centrifuge. The pellets were dissolved in 40 μl H 2 O and dried on speedvac again. The last procedure was repeated two more times. The final pellets were dissolved in 30 μl of electrophoresis buffer, pH 1.9, composed of 50 ml 88% formic acid, 156 ml glacial acetic acid and 1,794 ml H 2 O. A volume of 10 μl of each sample was mixed with 1 μl of unlabelled phosphor-amino acid standards, comprising 1.5 mg of each phospho-serine, phospho-threonine and phospho-tyrosine in total volume of 1 ml. The mixture of standards and labelled amino acids was spotted (in 0.5 ml aliquots) on the origin of a 20×20 cm glass backed cellulose thin-layer chromatography plate (Merck) and two samples originated from RBC cytosol and P. falciparum lysate were run in parallel in the first-dimension electrophoresis (pH 1.9) at 2000 V for 20–25 min in HTLE 7002 apparatus (Tony Hunter). The plate was air dried for 1 h before the second run was applied. The second-dimension electrophoresis buffer was composed of 100 ml glacial acetic acid, 10 ml pyridine, 10 ml 100 mM EDTA and 1,880 ml H 2 O, pH 3.5. For the second run the plate was rotated 90° counter-clockwise and the second-dimension electrophoresis was run at 1,800 V for 20 min. At the end of the run the plate was air dried for 1 h. To visualize the phospho-amino acid standards the plate was sprayed with 0.25% ninhydrin in acetone, then placed to the preheated oven (80–100 °C) for 5–10 min. Autoradiographs were performed in standard way by exposing at −80 °C overnight. Radioactive spots corresponding to phospho-amino acid standards were scrapped off from the plate and counted in scintillation counter. Ion-exchange fractionation of P. falciparum lysates Magnetic cell sorting-purified P. falciparum parasites pellets ( 32 P-labelled or 'cold') were resuspended in lysis buffer: 50 mM Tris, 0.5 mM EDTA, 5% β-glycerophosphate, pH7.6, supplemented with protease/phosphatase inhibitors (Roche) and 1% NP-40. Following incubation on ice for 10 min, the samples were centrifuged 3 min at 21,000 g (bench centrifuge) and the supernatants (in average 250–300 μl per medium pellet) were collected for further fractionation. Fractionation was carried out on an AKTA chromatographer (Amersham Pharmacia Biotec) using Resource Q (Amersham Pharmacia Biotec) anion-exchange columns (matrix volume 1 ml) in running buffer composed of 10 mM Tris, 5 mM EDTA and 20 mM β-glycerophosphate, pH7.4. The column batch was eluted with 1 M NaCl in a volume of 1 ml if the sample was going to be used in a tryptic digest. Alternatively, the proteins were eluted from the RQ column using a linear gradient of 0–1 M NaCl and 1 ml fractions were collected for use in experiments such as western blotting. To further prepare the samples for tryptic digestion, the pH of eluates was adjusted to 8–8.5 and treated, first, with 10 mM dithiothreitol in the presence 0.1% SDS for 30 min at room temperature to reduce disulphide bridges and, second, with 100 mM iodoacetamide for 1 h at room temperature (in dark) for alkylation of the reduced bonds. Trichloroacetic acid precipitation of the treated samples was performed by addition of 1 volume trichloroacetic acid stock (100% w/v) to 4 volumes of protein solutions. Samples were incubated on ice (10 min) and centrifuged at 21,000 g for 5 min. The pellets were washed once with ice-cold acetone (200 μl). After drying at room temperature the pellets were resuspended in 100 μl of 1% SDS in 50 mM triethylammonium bicarbonate (TEAB) buffer, pH 8.5 and finally diluted with 50 mM TEAB buffer, pH 8.5 to final volume 1 ml. If necessary, the samples were sonicated 3×5 s before making the final volume 1 ml. pH in the sample was adjusted to pH8–8.5. Tryptic digestion was carried out using agarose-immobilized trypsin (Thermo Scientific). Agarose beads were equilibrated before being used in an overnight digestion. The digested peptides were separated from the beads by centrifuging (1 min, 21 000 g ) and the supernatant was collected. The beads were washed with TEAB buffer 2×200 μl, and the supernatant and washes were combined. Digested samples were stored at −30 °C until use. Hydrophilic interaction chromatography Fractionation of digested peptides was performed on HPLC chromatographer (Hewlett Packard, 1100 Series) using TSKgel Amide-80 column, 4.6×250 mm, 5 mm particle size (Tosoh Bioscience). The column was equilibrated with a mixture of 80% Buffer B (98% acetonitrile, 0.1% TFA) and 20% Buffer A (98% H 2 O, 0.1% TFA) at flow rate 500 μl per min. Digested peptide solution was concentrated to about 100 μl on speedvac centrifuge and diluted with four parts of Buffer B. The precipitate which appeared in the solution after addition of acetonitrile was removed by centrifugation (5 min, 21,000 g ). Supernatant fraction was checked for pH and if necessary adjusted to pH 2.5–3.0 before applying to the column. The pellet was redissolved in a solution composed of 0.25 mM acetic acid, 30% (v/v) acetonitrile and used further for IMAC (see below). The supernatant fraction was loaded to the column in 80% Buffer B and eluted with decreasing gradient of acetonitrile as follows; (i) 0–5 min 80 % acetonitrile, (ii) 5–40 min 60% acetonitrile, (iii) 40–45 min 0% acetonitrile and (iv) 45–60 min 0% acetonitrile. Fractions (0.5 ml) were collected and directly used for immobilised metal affinity chromatography (IMAC) (see below). Enrichment of phosphopeptides PHOS-Select iron affinity gel (Sigma) was equilibrated with 5×1 ml IMAC load/wash buffer: 0.25 mM acetic acid, 30% (v/v) acetonitrile. A volume of 50 μl of 50% slurry of the resin was added directly to each 1 ml hydrophilic interaction liquid chromatography fraction. Samples were left on a rotating platform for 2 h at room temperature. Following incubation the fractions were transferred to the spin columns (MoBiTec GmbH) and centrifuged 30 s at 8,200 g . The flow-through (unbound peptides) were collected and concentrated on a speedvac centrifuge to small volume for further liquid chromatography-mass spectrometry (LC-MS)/MS analysis. The columns were washed twice with 200 μl of IMAC load/wash buffer and once with 200 μl of HPLC-grade H 2 O. Phospho-peptides bound to the resin were eluted with 2×100 μl solution composed of 0.4 M ammonium hydroxide, 30% (v/v) acetonitrile. The eluate was concentrated on a speedvac to a volume of 20 μl and analysed by LC-MS-MS analysis. The flow through from the IMAC resin was passed through a MonoTip TiO2 Pipette Tip columns (GL Sciences Inc) following the manufacturer's instructions. Peptides were eluted with 3.5% ammonia hydroxide and analysed by LC-MS/MS. The pellets which originated from insoluble in 80% acetonitrile peptide fraction (see above) were dissolved in IMAC load/wash buffer and the sample processed over the PHOS-Select iron affinity gel following the same protocol as described above. Parasite culture methods, antibody production, proteomic data analysis and mass spectrometry and protein analysis are described in the Supplementary Methods . Acccession codes: The proteomics data have been deposited on Tranche and can be accessed using the Tranche hash: JtHgFyh9HqIYMNWlXk2BTxav NlZutqY1fwalNMWAxEu7GmsuVFw0xQzUAuGf/3ZKgnXmZb33wtuawOhR33 cSO0QY2TsAAAAAAAAEvA==. How to cite this article: Solyakov, L. et al . Global kinomic and phospho-proteomic analyses of the human malaria parasite Plasmodium falciparum . Nat. Commun. 2:565 doi: 10.1038/ncomms1558 (2011).